Editing of human KV1.1 channel mRNAs disrupts binding of the N-terminus tip at the intracellular cavity In the nervous system, A→I RNA editing has an important role in regulating neuronal excitability. Ligand-gated membrane receptors, synaptic proteins, as well as ion channels, are targets for recoding by RNA editing. Although scores of editing sites have been identified in the mammalian brain, little is known about the functional alterations that they cause, and even less about the mechanistic underpinnings of how they change protein function. We have previously shown that an RNA editing event (I400 V) alters the inner permeation pathway of human K V 1.1, modifying the kinetics of fast inactivation. Here we show that the channel's inactivation gate enters deep into the ion permeation pathway and the very tip establishes a direct hydrophobic interaction with the edited position. By converting I to V, the intimacy of the interaction is reduced, allowing the inactivation gate to unbind with much faster kinetics. In excitable cells, precisely synchronized ionic currents generate the electric potentials that are the currency of communication. For the system to operate, the timing of turning the currents off is as important as the timing of turning them on. Accordingly, ion channels have developed intricate systems to switch off that override the signals to stay on, a process known as inactivation. In 1977 (ref. 1 ), without the aid of DNA sequences or structural data, Armstrong and Bezanilla proposed that inactivation of Na + currents in squid axon was caused by a tethered intracellular particle that would physically plug the channel's pore after it opened. Once sequence data became available, Aldrich and colleagues demonstrated the veracity of the ball and chain model using the shaker K V channel [2] , [3] . Further, they showed that the inactivation particle resides in the protein's cytoplasmic amino terminus. Across the spectrum of K + channels, the address of the inactivation particle varies. In some cases, like Shaker, it's part of the α subunit. In others, like human K V 1.1, it's part of an auxiliary β subunit. Not surprisingly, these inactivation machineries are subject to a vast and sophisticated set of posttranscriptional and posttranslational regulatory mechanisms [4] , [5] , [6] , [7] , including genetic recoding by RNA editing [8] , [9] , [10] , [11] . In rodent and human K V 1.1 channels, RNA editing recodes a highly conserved isoleucine to a valine (I400) [12] . This conversion is regulated in different regions of the nervous system [12] . Structural [13] and functional [14] data show that I400 is in the lining of the permeation pathway, in a region known as the channel's intracellular cavity. I400→V selectively targets the process of fast inactivation [8] , allowing edited channels to recover from inactivation about 20 times faster than their unedited counterparts. For a neuron, this change in function would greatly influence action potential shape, signal propagation and the firing pattern [15] , [16] , [17] , [18] , [19] , [20] . Here we investigate the precise mechanism by which I400V alters fast inactivation. The robust functional consequence of editing on inactivation is conserved in phylogenetically diverse K V channels, and mimicking I400V in Shaker K V channels (I470V) produces an increase in the speed of recovery from inactivation comparable to that seen in the human isoform [8] . Using an intracellular cysteine-less construct of shaker, we studied the mechanistic details underlying the I400V phenotype by changing the chemistry at this site by mutating it to a cysteine, and attaching different chemical moieties. Our results are consistent with the simple idea that nature uses RNA editing to increase the unbinding kinetics of the inactivation particle. It accomplishes this by selectively reducing the hydrophobic interaction between the tip of the amino terminus and its receptor, the edited codon within the intracellular cavity. Further, our experiments suggest that to obstruct permeation the inactivation particle must penetrate deeply into the intracellular cavity in an extended conformation. Intracellular cysteine-less channel construct Fast inactivation in Shaker K V channels is accomplished by a direct interaction between the N-terminal inactivation gate and the protein's permeation pathway [2] , [3] , [21] , [22] ( Fig. 1a ). Because position 470 lies deep within the inner vestibule of the permeation pathway, our overall goal was to define the specific position along the N terminus that interacts with it, and the chemical nature of the interaction. To accomplish the former, cysteines were engineered, in pairs, at position 470 and specific positions along the N terminus. For the latter, a single cysteine at codon 470 was modified with sulfhydryl reagents of different chemistries. As the inactivation gate transits towards its binding site, it likely interacts with different regions of the channel [23] , [24] , [25] . Therefore, sensible interpretations from our approach demand a channel construct that lacks cysteines at all other intracellular positions. 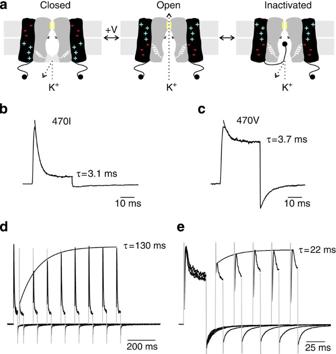Figure 1: Replicating the functional consequences of human KVchannel editing in a cysteine-less Shaker KVchannel background. (a) Cartoon representing the gating mechanisms of KVchannels. In response to a membrane depolarization, KVchannels open an intracellular gate that allows K+to permeate at rates near diffusion. Open channels can be directly blocked by an inactivating gate. (b) K+current from cysteine-less Shaker in response to a voltage step to +60 mV from a holding potential of −80 mV. All subsequent references to 'Shaker' refer to the cysteine-less background. Capacity transients were subtracted by a p/8 prepulse protocol. (c) Shaker I470V K+currents in response to an identical pulse protocol. This mutation mimics the RNA editing event (I400 V) in mammalian KV1.1 channels. Solid lines in (b,c) represent single exponential fits to the inactivation process. (d,e) Paired-pulse recovery from inactivation protocols of wild-type and I470 V Shaker KVchannels, respectively. Depolarizing pulses were to +60 mV and recovery was at −80 mV. Solid lines represent single exponential fits to the peak currents of the test pulses. The average recovery rate was 170±25 ms (n=9) for wild-type and 33±5 ms (n=6) for I470V channels. Capacity transients are shown in light gray. Figure 1: Replicating the functional consequences of human K V channel editing in a cysteine-less Shaker K V channel background. ( a ) Cartoon representing the gating mechanisms of K V channels. In response to a membrane depolarization, K V channels open an intracellular gate that allows K + to permeate at rates near diffusion. Open channels can be directly blocked by an inactivating gate. ( b ) K + current from cysteine-less Shaker in response to a voltage step to +60 mV from a holding potential of −80 mV. All subsequent references to 'Shaker' refer to the cysteine-less background. Capacity transients were subtracted by a p/8 prepulse protocol. ( c ) Shaker I470V K + currents in response to an identical pulse protocol. This mutation mimics the RNA editing event (I400 V) in mammalian K V 1.1 channels. Solid lines in ( b , c ) represent single exponential fits to the inactivation process. ( d , e ) Paired-pulse recovery from inactivation protocols of wild-type and I470 V Shaker K V channels, respectively. Depolarizing pulses were to +60 mV and recovery was at −80 mV. Solid lines represent single exponential fits to the peak currents of the test pulses. The average recovery rate was 170±25 ms ( n =9) for wild-type and 33±5 ms ( n =6) for I470V channels. Capacity transients are shown in light gray. Full size image Shaker K V channels contain four cysteines facing the intracellular side of the membrane: C96, C301, C308 and C505. Substituting the first three cysteines with serines and C505 with threonine (Methods) renders Shaker K V channels that inactivate and recover from inactivation similar to wild-type channels [8] , [25] , [26] ( Fig. 1b,d ). As with wild-type mammalian K V 1.1 and Shaker K V channels, mimicking the editing event in this background produces a comparable kinetic effect on inactivation [8] . Figure 1b,c show normalized current traces in response to a 30-ms depolarization to +60 mV from a holding potential of −80 mV for cysteine-less I470 and I470 V channels, respectively. The I470 V mutation greatly reduces the extent of inactivation, from about 80% to less than 30% ( Fig. 1b,c ), and speeds up the recovery from inactivation ( Fig. 1d,e ). From this, we conclude that mutating the four intracellular cysteines of Shaker K V channels does not interfere with the process of fast inactivation, nor does it alter the functional consequences that RNA editing has on it. Hydrophobicity at position 400 affects inactivation recovery When the edited position is substituted by a cysteine (I470C), the mutant channels inactivate to about 60% of the maximal current ( Fig. 2a ), and they recover with time constants of 30–50 ms ( Fig. 2c ; black open symbols). Clearly, both the on-and-off kinetics of I470C are different from wild-type channels. This is expected. As nature has shown with the editing event itself, even small changes to the side chain at this position can have large affects on inactivation [8] . Next, we took advantage of sulfhydryl reagents to attach specific moieties to I470C through a disulfide linkage. When a single methyl group was added to position 470 with MMTS, the channels did not lose their ability to open, inactivate and close in response to voltage ( Fig. 2b ). Interestingly, the steady-state level of inactivation increased to about 90% ( Fig. 2b ) and the recovery from inactivation was slowed down about 25 fold, from 53 ms ( Fig. 2c ; black open circles) to 1.4 s ( Fig. 2c ; red filled circles). These results suggest that increasing the hydrophobicity of the cavity stabilizes a bound inactivation particle. 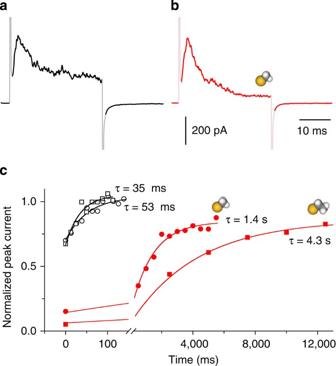Figure 2: Modification of Shaker KVI470C channels with hydrophobic MTS reagents. (a,b) K+current traces recorded from the same population of Shaker KVchannels before (a) and after (b) complete modification with MMTS, which adds a methyl group. Capacity transients are depicted in light tones. (c) Time courses of recovery from inactivation before (open symbols) and after (filled red symbols) complete modification with MMTS (circles) or EMTS, which adds an ethyl group (squares). Solid lines represent single exponential fits. Average fold changes after modification were 63±5 for MMTS (n=4) and 190±50 (n=4) for EMTS. Figure 2c (open and red filled squares) shows another experiment where the channels were modified with EMTS, a reagent that adds an ethyl moiety. In this case, recovery from inactivation was slowed to an even greater extent, with a time constant more than 100-fold slower than before the modification. These results imply that as the intracellular cavity becomes more hydrophobic after modification, a bound inactivation gate establishes a much stronger hydrophobic interaction, resulting in a slower OFF rate from inactivation. Figure 2: Modification of Shaker K V I470C channels with hydrophobic MTS reagents. ( a , b ) K + current traces recorded from the same population of Shaker K V channels before ( a ) and after ( b ) complete modification with MMTS, which adds a methyl group. Capacity transients are depicted in light tones. ( c ) Time courses of recovery from inactivation before (open symbols) and after (filled red symbols) complete modification with MMTS (circles) or EMTS, which adds an ethyl group (squares). Solid lines represent single exponential fits. Average fold changes after modification were 63±5 for MMTS ( n =4) and 190±50 ( n =4) for EMTS. Full size image Even though the previous results suggest that hydrophobic interactions within the intracellular cavity stabilize a bound inactivation gate, they do not rule out the possibility that steric rather than hydrophobic interactions determine the OFF rate from inactivation. To address this issue, we attached polar residues to I470C that are about the same size as an ethyl group. 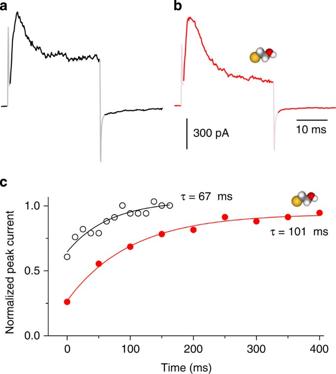Figure 3: Modification of Shaker KVI470C channels with polar reagents. (a,b) K+current traces recorded from the same population of Shaker KVchannels before (a) and after (b) complete modification with MTSHE, which adds a hydroxyethyl group. Capacity transients are depicted in light tones. (c) Time courses of recovery from inactivation before (open circles) and after (filled red circles) complete modification with MTSHE. Solid lines represent single exponential fits. Average fold change after modification was 3±1 (n=4). Figure 3 shows an example using MTSHE, a reagent that attaches a hydroxyl ethyl group. Before modification, the channels inactivated to ~50% of the maximal current ( Fig. 3a ). After complete modification, they inactivated slightly more, to about 75% ( Fig. 3b ). They also recovered from inactivation slightly more slowly than untreated channels, with a time constant of ~100 ms ( Fig. 3c ). Similar results were also observed with MTSCM, a reagent that adds a carboxy methyl group (data not shown). These results suggest that steric factors have a relative minor role in the mechanism by which RNA editing alters the process of fast inactivation, and most of the changes in unbinding kinetic by the I to V conversion are determined by hydrophobic interactions between the inactivation gate and the edited position. Figure 3: Modification of Shaker K V I470C channels with polar reagents. ( a , b ) K + current traces recorded from the same population of Shaker K V channels before ( a ) and after ( b ) complete modification with MTSHE, which adds a hydroxyethyl group. Capacity transients are depicted in light tones. ( c ) Time courses of recovery from inactivation before (open circles) and after (filled red circles) complete modification with MTSHE. Solid lines represent single exponential fits. Average fold change after modification was 3±1 ( n =4). Full size image Next, we tested how the recovery rate from inactivation relates to the degree of hydrophobicity at position 470. There are four natural aliphatic amino acids: Ala, Val, Leu and Ile. The side chains of these amino acids have no reactive groups, so they can only establish hydrophobic interactions. 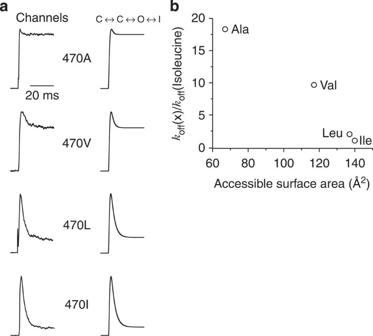Figure 4: Effect of different aliphatic residues at position 470 on inactivation. (a) The left column shows single-current traces from Shaker KVchannels with different aliphatic amino acids at position 470. All currents are in response to a voltage step to +60 mV from a holding potential of −80 mV. The right column shows four simulations using the simple kinetic scheme shown on top. Onlykoffof the transition O↔I was varied. It was 550, 290, 60 and 30 s−1for Ala, Val, Leu and Ile, respectively. The forward rate for O↔I was 300 s−1. The remaining C↔C↔O transitions have forward rates of 700 s−1times a Boltzmann factor and backward rates of 1 s−1times a Boltzmann factor. (b) The plot correlates the simulated fold change inkoffcaused by a particular mutation at I470 with the accessibility surface area of the mutant side chain. Figure 4a shows an example of a current record in response to a 30 ms depolarization to +60 mV for each of the aliphatic residues substituted at position 470. The right column shows four simulations using a simple kinetic scheme (top). The only difference between these simulations is the unbinding rate constants: k off Ala=550 s −1 , k off Val=290 s −1 , k off Leu=60 s −1 and k off Ile=30 s −1 . The changes in unbinding kinetics correlate well with the accessible surface area of the side chains ( Fig. 4b ). These results, combined with those presented in earlier figures, strongly support the idea that the inactivation gate establishes a hydrophobic interaction with the intracellular cavity, and that I470 is a major contributor to this interaction with its side chain largely determining the unbinding kinetics. Figure 4: Effect of different aliphatic residues at position 470 on inactivation. ( a ) The left column shows single-current traces from Shaker K V channels with different aliphatic amino acids at position 470. All currents are in response to a voltage step to +60 mV from a holding potential of −80 mV. The right column shows four simulations using the simple kinetic scheme shown on top. Only k off of the transition O↔I was varied. It was 550, 290, 60 and 30 s −1 for Ala, Val, Leu and Ile, respectively. The forward rate for O↔I was 300 s −1 . The remaining C↔C↔O transitions have forward rates of 700 s −1 times a Boltzmann factor and backward rates of 1 s −1 times a Boltzmann factor. ( b ) The plot correlates the simulated fold change in k off caused by a particular mutation at I470 with the accessibility surface area of the mutant side chain. Full size image Interactions of the N terminus with the intracellular cavity In their pioneering studies [2] , [3] , Aldrich's group established that fast inactivation in K V channels originates from the interactions between the N terminus and the core of the protein. The inactivation gate (N-terminus) resembles an open channel blocker [26] that can compete with potassium channel inhibitors, like TEA [27] . Even though each Shaker K V channel has four N termini, one is sufficient to produce inactivation [28] , [29] . Further, it has been proposed that the receptor site for the inactivation particle is the intracellular cavity of the channel [24] . As shown here, the most plausible mechanism, by which RNA editing in human K V channels alters fast inactivation, is by a change in the unbinding kinetics of the inactivation gate. Because hydrophobic interactions have a determining role in this process, we anticipated a close intimacy between specific amino acids at the N-terminus and position 470. To explore this possibility, we developed a series of double cysteine mutants, one at the edited position (I470C) and the other at positions 2 through 7 along the N-terminus of the channel. If any of the N-terminal cysteines closely interact with I470C, located deep at the intracellular cavity, we would expect the formation of a disulphide bond, resulting in a current reduction that would not recover on repolarization. I470C channels with cysteines also at positions 3 through 7 produced functional proteins that activated in response to depolarization, and inactivated to different extents. However, none showed signs of an irreversible current reduction after repetitive stimulation ( Supplementary Fig. S1a ). Thus positions 3–7 do not appear to make contact with position 470. Examining position 2 was more difficult. The double mutant 2C-470C did not efficiently reach the cell surface. Fluorescence emitted from C-termini GFP fusion constructs showed that this mutant was retained intracellularly ( Supplementary Fig. S1b ). To overcome this impediment, we coexpressed channel constructs with either a cysteine at position 2 or at 470. The A2C channels responded normally to voltage and did not show any signs of disulfide bond formation between cysteines at position 2 on neighbouring subunits ( Supplementary Fig. S2 ). By co-transfecting both constructs, we would expect heterotetramers to form [29] , each channel containing some cysteines at both positions, and homotetramers of A2C and I470C. On patch excision, ionic currents through mixed channels diminished irreversibly ( Fig. 5 ; filled black symbols), presumably by the formation of disulfide bonds between cysteines at positions 2 and 470. A minor amount of ionic current remained, likely through homotetrameric channels. By exposing the patch to mercaptoethanol, we were able to recover the ionic currents ( Fig. 5 ; filled red symbols), indicating that the initial irreversible current reduction was caused by disulfide bond formation in heterotetramers between 2C and 470C. These results show that the tip of the N terminus (position 2) is able to enter deeply into the intracellular cavity, at least as far as position 470. 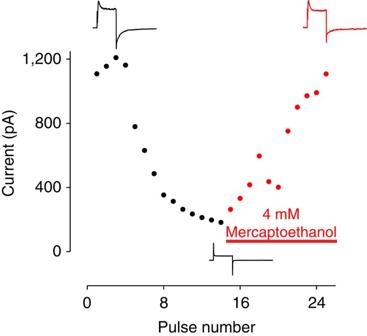Figure 5: Disulfide bridges between the tip of the N terminus and the intracellular cavity. Filled circles represent the average steady-state current amplitude (last 10 ms) of consecutive 30 ms depolarizations to +60 mV performed every 5 s. The first symbol corresponds to the first pulse after the patch was excised from the cell. To illustrate reversibility by mercaptoethanol, three current records are shown: one soon after excision, one after substantial oxidation, immediately before application of mercaptoethanol, and another after full recovery. We observed similar results in 8 inside–out excised patches. Figure 5: Disulfide bridges between the tip of the N terminus and the intracellular cavity. Filled circles represent the average steady-state current amplitude (last 10 ms) of consecutive 30 ms depolarizations to +60 mV performed every 5 s. The first symbol corresponds to the first pulse after the patch was excised from the cell. To illustrate reversibility by mercaptoethanol, three current records are shown: one soon after excision, one after substantial oxidation, immediately before application of mercaptoethanol, and another after full recovery. We observed similar results in 8 inside–out excised patches. Full size image As more RNA editing events are uncovered, and their functional consequences elucidated, we are beginning to understand how functional diversity is created by this mechanism. In contrast, we are virtually ignorant of the rules that nature uses to accomplish these changes in protein function. In fact, RNA editing within the permeation pathway of GluR2 receptors is the only example where we know the precise mechanism used to alter protein function [30] , [31] . In this case, a change in the intrinsic electrostatic potential of the pore impedes Ca 2+ permeation through the channel. Here we show that RNA editing reduces a hydrophobic interaction between the cytoplasmic inactivation gate and it's receptor within the channel's core. The removal of a single methyl group destabilizes this interaction sufficiently to permit the inactivation gate to unbind ~20 times faster. Our data clearly shows that the interaction is hydrophobic in nature, and its interruption is not due to steric factors. Furthermore, the position of the edited codon gives us further clues about how the process of fast inactivation works. To understand how ion flow through a K V channel can be stopped, it is useful to consider the entire permeation pathway ( Fig. 6 ). To leave the cell, intracellular K + , driven by concentration and electrical gradients, enter the channel through four symmetrical portholes, oriented parallel to the membrane surface. These openings, formed by the top of the T1 domain and the bottoms of the inner helices, are large, ~20 Å in diameter ( Fig. 6a ). After passing through them, the ions go through the open activation gate and enter into the internal vestibule, bounded on the sides by the S6 helices, and on the top by the partial pore helices ( Fig. 6b ). This inner vestibule resembles a long cylinder, somewhat wider at top, with a diameter of about 15 Å. The entrance into the narrow selectivity filter is at the top of the inner vestibule. Here the permeation pathway constricts to about 6 Å and after passing through it, the ions reach the extracellular side. Ever since the seminal papers of Armstrong [32] and Aldrich [2] , [3] , [21] , [22] , it has been generally agreed that inactivation by quaternary ammonium derivatives, and the N-terminal inactivation gate occurs by direct physical block to a common site [24] , [26] , [27] . 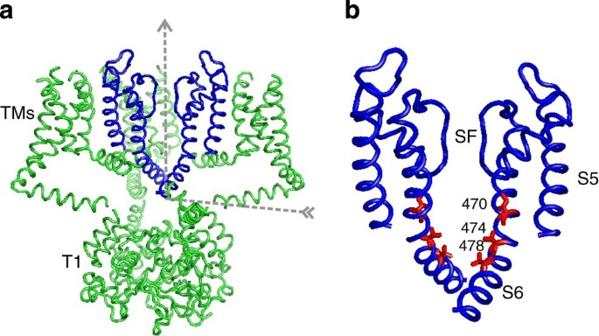Figure 6: Cartoon view of the rat KV1. 2 structure. The figure comes from PDB 2A79 (MMDB ID: 34,400). (a) View of the α subunit tetramer. T1, tetramerization domain; TM, transmembrane helices. The arrow marks the route of K+flow through the channel. For clarity, S1–S6 has been removed from the subunit in the foreground, and S5–S6 has been removed from the subunit in the background. (b) View of the inner vestibule. Only S5–S6 (with the intervening pore helices) from 2 subunits are shown. Numbering of V478, V474 and I470 corresponds to the Shaker KVchannel's sequence. SF, selectivity filter. S5–S6 is shown in blue and the rest of the channel in green. Figure 6: Cartoon view of the rat K V 1. 2 structure. The figure comes from PDB 2A79 (MMDB ID: 34,400). ( a ) View of the α subunit tetramer. T1, tetramerization domain; TM, transmembrane helices. The arrow marks the route of K + flow through the channel. For clarity, S1–S6 has been removed from the subunit in the foreground, and S5–S6 has been removed from the subunit in the background. ( b ) View of the inner vestibule. Only S5–S6 (with the intervening pore helices) from 2 subunits are shown. Numbering of V478, V474 and I470 corresponds to the Shaker K V channel's sequence. SF, selectivity filter. S5–S6 is shown in blue and the rest of the channel in green. Full size image Where along the permeation pathway does the inactivation particle block ion flow? The portals leading into the inner vestibule are not good candidates because there are four of them and a single inactivation particle is all that is required to produce block [29] . It is more reasonable to hypothesize that the inactivation particle binds within the inner vestibule. To stop current flow in this chamber, it would have to adopt a tertiary structure so that ion flow around it would be restricted. Alternatively, it could reach the top of the chamber and plug the narrow entrance to the selectivity filter. Previous functional studies suggest that the inactivation particle does not adopt an ordered structure [22] , and that it enters the inner vestibule in an extended configuration [24] . In fact, by applying a mutant cycle analysis, Zhou et al . [24] predicted specific interactions between the inactivation particle of the human K V β1.1 and the hydrophobic surface at the bottom of the inner vestibule of K V α1.4. They suggested that position 3 of the inactivation particle binds to the equivalent of V474 and V478 from this study. Our data supports this idea and extend it. By demonstrating that position 2 of the inactivation particle interacts with I470, we show that this structure reaches near the top of the inner vestibule and that its tip is positioned close to the entrance of the selectivity filter, supporting the idea that block occurs at this site. Unlike most regulatory mechanisms that act on the level of expression, RNA editing can fine tune protein function. By changing an adenosine to an inosine, 16 different amino acids can be recoded, lending a powerful set of tools for the process to exploit. For example, single amino acid changes, caused by editing, alter the function of serotonin receptors [33] , K V channels [8] , [9] , [10] , [11] , [34] , Na + channels [35] , GABA A receptors [36] , Na + /K + -ATPase [37] , and ADARs themselves [38] . Our data extends these studies by providing a mechanistic interpretation of how an amino-acid change, caused by editing, renders its effect. The removal of a single methyl group drastically, and specifically, targets the unbinding of the K V inactivation particle from its receptor [8] . Further, we showed that once the intracellular cavity has lost a methyl group, it loses an important hydrophobic interaction with the tip of the N terminus that likely enters deep into the cavity in an extended conformation. Interestingly, this same editing site can modulate the binding of hydrophobic drugs that interact with the intracellular cavity [39] . From a neurophysiological perspective, we would predict that the I400 V change would enable a neuron to sustain much faster firing rates. It is worth noting that this edit is most frequent in the medulla, thalamus and spinal cord [12] , regions that contain neurons with some of the fastest firing rates documented [40] , [41] , [42] , [43] , [44] , [45] , [46] . A finer scale study of this edit's expression will help support the idea that it directly regulates firing rates. Selection of K V channel background Several reasons prompted us to perform this study using the Shaker K V channel as a background. First, in hK V 1.1 channels the inactivation gate is part of an auxiliary intracellular β subunit [47] . In contrast, the inactivating particle in Shaker K V channels comes from the N terminus of the same α subunit that forms the channel, and, therefore, we only needed to concern ourselves with expression of a single protein. Second, N-type inactivation in hK V 1.1 is highly regulated by a variety of cellular processes [4] , [5] , [6] , complicating mechanistic interpretations. Third, between α and β subunits of hK V 1.1 channels there are fifteen cysteines, whereas in Shaker there are only seven, of which only four face the intracellular environment. Our previous experience in working with these four cysteine residues in the context of methanethiosulfonate modification experiments [14] , [23] allowed us to more efficiently define specific experimental constructs and conditions. In this study, we attempted a series of experiments to functionally detect cross-linking between two cysteines facing the intracellular side of the channel: one at the N terminus of the protein and the second within the intracellular cavity of the channel. Therefore, we needed to find an appropriate background with no intracellular cysteines that also expresses robustly in HEK293 cells. Shaker K V channel possesses intracellular cysteines at positions 96, 301, 308 and 505. Previously [23] , we found that when these four cysteines are substituted by serine and valine (C96S, C301S, C308S and C505V), the channels expressed very well. However, when extra mutations to cysteines were made in this background, they sometimes expressed poorly. From a variety of experiments, we determined that C96S and C505V are the culprits. We undertook a systematic effort to find mutants at these two sites that did not hinder expression. We found that mutations C96S and C505T (in the context of I470C, C301S, C308S) resulted in channels that express well. All experiments were performed with this construct. Mutagenesis and transfection All mutations were made using mutagenic oligonucleotides and standard PCR techniques. The integrity of the constructs was checked by sequencing. For expression, shaker channels were subcloned into the expression vector GW1-CMV (British Biotechnology) and transiently expressed in HEK393 cells (ATCC). Expression plasmid (25–35 μg) was co-transfected with 1 μg πH3-CD8 and highly transfected cells were detected with CD8 antibody-coated beads [48] (Dynal). Transfections were performed with a Gene Pulser II electroporator (Bio Rad) using standard setting. Electrophysiological recordings All electrophysiological experiments were performed using inside–out patches [49] excised 2–4 days after DNA transfection. Voltage control and current acquisition was achieved with a Digidata 1322A (Molecular Devices) board, an Axopatch 200b patch clamp (Molecular Devices) and Clampex Software (Molecular Devices). Ionic currents were sampled at 5 kHz and filtered at 2 kHz. Recording electrodes were made from borosilicate glass and had a resistance of ~2 MΩ. The internal solution contained (in mM): 160 KCl, 1 EGTA, 10 HEPES (pH=7.4). Mg 2+ was removed because we have previously found that the I470C mutation renders intracellular Mg 2+ a voltage-dependent blocker [50] . The external solution contained (in mM): 150 NaCl, 10 KCl, 3 CaCl 2 , 1 MgCl 2 , 10 HEPES (pH=7.4). All salts were acquired from FLUKA (puriss grade). EGTA and HEPES were obtained from SIGMA. GFP fluorescence imaging Cysteine-less Shaker coding sequences (WT and A2C-I470C) were subcloned in frame into the pAcGFP1-N2 vector (Clontech). 30 μg of plasmid DNA were transfected by electroporation into HEK293 cells. After 24 h cells were fixed with 3.4% paraformaldehyde (Electron Microscopy Sciences) and imaged using a Zeiss LSM 510 confocal microscope. How to cite this article: Gonzalez, C. et al . Editing of human K V 1.1 channel mRNAs disrupts binding of the N-terminus tip at the intracellular cavity. Nat. Commun. 2:436 doi: 10.1038/ncomms1446 (2011).